Shared active site architecture between archaeal PolD and multi-subunit RNA polymerases revealed by X-ray crystallography Archaeal replicative DNA polymerase D (PolD) constitute an atypical class of DNA polymerases made of a proofreading exonuclease subunit (DP1) and a larger polymerase catalytic subunit (DP2), both with unknown structures. We have determined the crystal structures of Pyrococcus abyssi DP1 and DP2 at 2.5 and 2.2 Å resolution, respectively, revealing a catalytic core strikingly different from all other known DNA polymerases (DNAPs). Rather, the PolD DP2 catalytic core has the same ‘double-psi β-barrel’ architecture seen in the RNA polymerase (RNAP) superfamily, which includes multi-subunit transcriptases of all domains of life, homodimeric RNA-silencing pathway RNAPs and atypical viral RNAPs. This finding bridges together, in non-viral world, DNA transcription and DNA replication within the same protein superfamily. This study documents further the complex evolutionary history of the DNA replication apparatus in different domains of life and proposes a classification of all extant DNAPs. In all forms of cellular life, DNA polymerases (DNAPs) play central roles in genome replication, maintenance and repair, and have therefore been the subject of intensive research for decades [1] . Over the years, all DNAPs have been grouped in different families, using sequence alignments [2] , [3] : PolA, PolB, PolC, PolD, PolX, PolY and reverse transcriptases. Strikingly, nearly all of them belong to one of two different folds [4] , the Klenow-fold (PolA, PolB, PolY and reverse transcriptases) or the Polβ-fold (PolC and PolX). The only class of DNA polymerases left whose structure is unknown and for which the catalytic domain has no assigned fold is PolD. PolD exists in all Archaea, except Crenarchaea, and is a replicative polymerase responsible for initiating DNA synthesis at both leading and lagging strands [5] , [6] , [7] , [8] . It is composed of a large catalytic subunit (DP2) and a smaller subunit with 3′–5′ proofreading exonuclease activity (DP1) [5] . Apart from the N-terminal regions of its DP1 (ref. 9 ) (1–50) and DP2 (ref. 10 ) (50–280) subunits, neither the structure of the catalytic polymerase nor the one of the exonuclease domain has been determined yet. While DP1 is known to belong to the calcineurin-like phosphodiesterase superfamily [11] , DP2 shows no sequence similarity to other proteins with the exception of a short C-terminal zinc-binding motif in eukaryotic Polɛ (ref. 12 ). To help resolve the uncertainty concerning the evolutionary origins of D-family DNAP, we determined the crystal structures of two large fragments of both DP1 and DP2 subunits of the Pyrococcus abyssi PolD. Crystallization of both DP1 and DP2 catalytic subunits The structure of DP1 presented here encompasses amino acids 144–622, leaving out a flexible N-terminal region that is not evolutionary conserved and not needed for exonuclease activity ( Fig. 1a ). The DP2 construct covers amino acids 1–1,050 from DP2 DNAP subunit, leaving out a C-terminal domain (CTD; 1,051–1,270) dedicated to interaction with DP1 (refs 13 , 14 ; Fig. 1b ). While the interaction between the two subunits is essential for the full activity of PolD [7] , [14] , [13] , both DP1 and DP2 constructs described here are capable of digesting mispaired 3′–5′ nucleotides and of extending a DNA primer in a templated manner, respectively ( Supplementary Fig. 1 ). Both DP1 and DP2 crystal structures were determined individually by experimental phasing and refined at final resolutions of 2.5 and 2.2 Å, respectively. 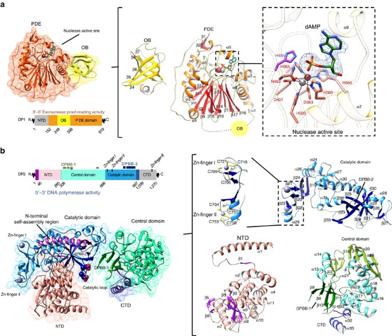Figure 1: Overview of DP1 and DP2 structures. (a) Left: cartoon representation of DP1 (144–622) coloured according to domains: PDE domain, orange; OB domain, yellow. Deleted regions, absent from the construct that was crystallized, are shown in grey. Centre: enlarged views of individual OB and PDE domains coloured by secondary structure. Right: structural details of the DP1 exonuclease active site. Catalytic residues and dAMP are shown as sticks. The blue mesh shows the Fo–Fc omit map electron density surrounding dAMP contoured at 3.0σ. (b) Left: cartoon representation of DP2 (1–1,050) coloured according to domains: N-terminal self-assembly region, purple; NTD, pink; central domain, cyan; catalytic domain, blue; CTD, dark blue. The aspartic side chains of the conserved D956 and D958 catalytic residues are shown as spheres. Deleted regions, absent from the construct that was crystallized, are shown in grey. Right: enlarged views of individual DP2 domains coloured by secondary structure. Zn2+ions are shown as spheres, and side chains of the cysteine-coordinating residues are shown as sticks. Figure 1: Overview of DP1 and DP2 structures. ( a ) Left: cartoon representation of DP1 (144–622) coloured according to domains: PDE domain, orange; OB domain, yellow. Deleted regions, absent from the construct that was crystallized, are shown in grey. Centre: enlarged views of individual OB and PDE domains coloured by secondary structure. Right: structural details of the DP1 exonuclease active site. Catalytic residues and dAMP are shown as sticks. The blue mesh shows the Fo–Fc omit map electron density surrounding dAMP contoured at 3.0 σ . ( b ) Left: cartoon representation of DP2 (1–1,050) coloured according to domains: N-terminal self-assembly region, purple; NTD, pink; central domain, cyan; catalytic domain, blue; CTD, dark blue. The aspartic side chains of the conserved D956 and D958 catalytic residues are shown as spheres. Deleted regions, absent from the construct that was crystallized, are shown in grey. Right: enlarged views of individual DP2 domains coloured by secondary structure. Zn 2+ ions are shown as spheres, and side chains of the cysteine-coordinating residues are shown as sticks. Full size image Structure of the PolD DP1 proofreading exonuclease subunit DP1 structure shows an insertion of an oligonucleotide/oligosaccharide binding (OB) domain in the N-terminal region of the large calcineurin-like phosphodiesterase (PDE) domain ( Fig. 1a ). The OB domain (residues 249–338) consists of a five-stranded β-barrel (β 4 –β 8 ) wrapped around by helix α 2 on one side. The PDE domain (residues 152–248 and 339–619) comprises a two-layer β-sheet (β 3 , β 13 –β 17 , and β 9 –β 12 , β 18 –β 19 , respectively) flanked by α-helices α 3 –α 6 on one side, and by α-helices α 7 –α 8 on the other side. The PDE domain contains five conserved phosphodiesterase motifs, which form the nuclease active site ( Fig. 2a and Supplementary Fig. 2 ). These motifs are located in loops connecting the core β-strands together and with their flanking α-helices. These loops converge to form a solvent-exposed active site that contains two metal ions, modelled as Fe 3+ and Zn 2+ based on anomalous maps using diffraction data measured at the Fe and Zn edges, respectively ( Fig. 1a and Supplementary Fig. 3 ). Metal ions are tetrahedrally coordinated by seven conserved residues distributed in several phosphodiesterase motifs (D363, H365, D407, N453, H500, H563 and H565; Fig. 1a and Supplementary Fig. 4 ). The oxidation state of the iron ion was modelled as Fe 3+ based on the fact that the metal-coordination geometry observed in DP1 closely resembles that of di-metal (Fe 3+ /Zn 2+ ) phosphatases, including mammalian calcineurin [15] , and the kidney bean purple acid phosphatase [16] . Furthermore, Fe 3+ has been shown to be required for calcineurin, a structurally similar hydrolase, which undergoes a loss of activity on reduction of Fe 3+ into Fe 2+ (ref. 17 ). 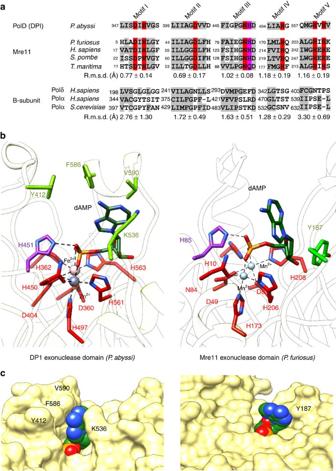Figure 2: Structure of the DP1 nuclease active site. (a) Structure-based alignment of the six most conserved phosphoesterases motifs of the PolD DP1 subunit, with representative structures of Mre11 ((PDBid: 1II7)P. furiosus19, (PDBid: 3T1L)Homo sapiens67, (PDBid: 4FBW)Schizosaccharomyces pombe68and (PDBid: 3THO)Thermotoga maritima69), and eukaryotic regulatory B-subunits ((PDBid: 3EOJ)H. sapiensPolδ (ref.26, PDBid: 4Y97)H. sapiensPolα (ref.27, PDBid: 3FLO)S. cerevisiaePolα (ref.70). The values indicated below the alignments indicate the r.m.s.d. (in Å) measured on Cα atoms, after superposing each structure on DP1. The r.m.s.d. values are averaged separately for the Mre11 and eukaryotic regulatory B-subunits subgroups of structures. Metal-coordinating residues and the catalytic proton-donor residue are highlighted in red and purple, respectively. (b) Comparison of the DP1 andP. furiosusMre11 (PDBid: 1II7 (ref.19)) nuclease active sites. Metal-coordinating residues (red), proton-donor catalytic residue (purple), dAMP (dark green) and nucleotide base-binding residues (light green) are shown as sticks. (c) Compared solvent-accessible surface of the DP1 andP. furiosusMre11 nuclease active sites. The dAMP molecule is in CPK-sphere representation. Figure 2: Structure of the DP1 nuclease active site. ( a ) Structure-based alignment of the six most conserved phosphoesterases motifs of the PolD DP1 subunit, with representative structures of Mre11 ((PDBid: 1II7) P. furiosus [19] , (PDBid: 3T1L) Homo sapiens [67] , (PDBid: 4FBW) Schizosaccharomyces pombe [68] and (PDBid: 3THO) Thermotoga maritima [69] ), and eukaryotic regulatory B-subunits ((PDBid: 3EOJ) H. sapiens Polδ (ref. 26 , PDBid: 4Y97) H. sapiens Polα (ref. 27 , PDBid: 3FLO) S. cerevisiae Polα (ref. 70 ). The values indicated below the alignments indicate the r.m.s.d. (in Å) measured on Cα atoms, after superposing each structure on DP1. The r.m.s.d. values are averaged separately for the Mre11 and eukaryotic regulatory B-subunits subgroups of structures. Metal-coordinating residues and the catalytic proton-donor residue are highlighted in red and purple, respectively. ( b ) Comparison of the DP1 and P. furiosus Mre11 (PDBid: 1II7 (ref. 19 )) nuclease active sites. Metal-coordinating residues (red), proton-donor catalytic residue (purple), dAMP (dark green) and nucleotide base-binding residues (light green) are shown as sticks. ( c ) Compared solvent-accessible surface of the DP1 and P. furiosus Mre11 nuclease active sites. The dAMP molecule is in CPK-sphere representation. Full size image Structure of the PolD DP1-dAMP complex Among the calcineurin-like superfamily of proteins, DP1 shows the highest structural similarity with the Mre11 exo-/endonuclease, a key player in DNA repair [18] . To gain insight into the catalytic exonuclease mechanism of PolD, DP1 was co-crystallized together with deoxy-adenosine monophosphate (dAMP) that mimics the 3′-end of the DNA being digested ( Figs 1a and 2b ). This allows a detailed comparison with the active site of Pyrococcus furiosus Mre11 that was also solved in complex with dAMP [19] ( Fig. 2b ). P. abyssi DP1 and P. furiosus Mre11 PDE domains superimpose well (root mean square deviation (r.m.s.d.) value of 2.21 Å calculated over 157 residues; Supplementary Fig. 5 ) and their metal ions coordinating residues are remarkably conserved ( Fig. 2a and Supplementary Fig. 4 ). Consistent with what is observed from other ligand-bound PDE structures, dAMP binds mainly via interactions between its phosphate moiety and the coordinated metals, in both P. furiosus Mre11 (ref. 19 ) and DP1 structures ( Fig. 2b ). The phosphate moiety also interacts with a conserved histidine residue, H85 in Mre11 (ref. 20 ) and H451 in DP1 (ref. 21 ), which has been shown to be essential for nuclease activity for re-protonating the 3′-OH of the leaving DNA. These observations suggest that DP1 shares the canonical hydrolase mechanism where the metal ions activate the attacking hydroxide ion, which catalyses hydrolysis of the phosphodiester bond [22] . However, interactions with the adenine base moiety are markedly different between DP1 and P. furiosus Mre11. In Mre11, the adenine base of dAMP has little interaction with active site residues, except for a base-stacking interaction with the side chain of Y187 ( Fig. 2b ) [19] . The Mre11 active site thus exposes the Watson–Crick face of the purine moiety ( Fig. 2c ), suggesting that the 3′-terminal base is recognized intra-helically [19] , as expected for a nuclease capable of 3′–5′ digestion on paired nucleotides of a 3′-recessed DNA [23] . In contrast to Mre11, the adenine base binds into a narrow groove of the DP1 active site, contributed by the β 8 –α 5 loop and α-helix α 9 from one side, and the α 8 –β 13 loop and α-helix α 7 from the other side. The adenine base mainly binds through hydrophobic interactions with the side chains of Y415, V593, F589 and the alkyl moiety of K536 ( Fig. 2c ). As expected for a non-selective nuclease, these residues do not show specific interactions with the adenine base, but instead define a pocket that partially masks the Watson–Crick face of the bound nucleotide ( Fig. 2c ). This observation provides a structural rationale to biochemical assays showing that DP1 exonuclease prefers mispaired nucleotides over paired nucleotides [24] . The observed preference of PolD DP1 for mispaired nucleotides at the 3′-end is characteristic for a DNAP-associated proofreading exonuclease. Evolutionary relationships to eukaryotic DNAPs B-subunits Consistent with bioinformatics predictions [11] , results of a Dali [25] search of the protein data bank ( Supplementary Fig. 6 ) show that DP1 shares the strongest overall structural similarity with the regulatory B-subunits of the eukaryotic Polδ (ref. 26 ) and Polα (ref. 27 ; Fig. 3 ). DP1 and the B-subunit of Polδ show a remarkable degree of three-dimensional structural similarity (r.m.s.d. value of 2.56 Å calculated over 322 residues). The region of conservation encompasses both OB (r.m.s.d. value of 1.64 Å calculated over 66 residues) and PDE (r.m.s.d. value of 2.28 Å calculated over 257 residues) domains. However, despite the conserved overall architecture, all DP1 catalytic residues are lost in eukaryotic B-family regulatory subunits ( Fig. 2a ). In Polδ and Polɛ, the 3′–5′ proofreading activity and DNA polymerizing activities are provided instead by their large A-catalytic subunit, which contains an exonuclease domain. It is noteworthy that the exonuclease domains of Polδ and Polɛ are structurally distinct from that of DP1 and the calcineurin-like PDE superfamily. In addition to their PDE domains, comparison of DP1 and eukaryotic B-subunit OB domains also show substantial structural differences that might account for functional ones. Interestingly, when used in database searches on its own, DP1 OB domain has stronger structural similarity with OB domains of class II-b aminoacyl-tRNA synthetases [28] and RPA, a DNA single-stranded binding protein involved in replication [29] , rather than with OB domains of eukaryotic B-subunits ( Supplementary Fig. 6 ). The OB-fold architecture displays a conserved binding face well adapted to interact both with RNA and ssDNA [30] , which is also present in DP1 but altered in eukaryotic DNAP B-subunits. Indeed, the surface of DP1 OB domain shows a positive electrostatic potential patch that occupies a location similar to the DNA-binding face observed in other OB domains [30] ( Fig. 3 ). Polδ and Polα OB domains display no such clusters of conserved positively charged residues suggesting that their oligonucleotides’ binding properties are altered. 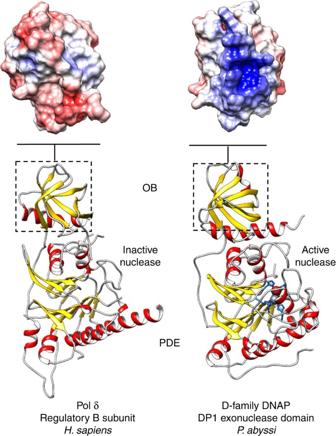Figure 3: Evolutionary relationships of DP1 to eukaryotic DNAPs B-subunits. Ribbon diagrams highlighting the shared architecture between PolD DP1 andHomo sapiensPolδ B-subunit (PDBid: 3EOJ (ref.26)). Top panels show the electrostatic potentials of DP1 and Polδ OB domains mapped on their solvent-accessible surface at contouring ±5 kT e−1. The potential was calculated with APBS64. Figure 3: Evolutionary relationships of DP1 to eukaryotic DNAPs B-subunits. Ribbon diagrams highlighting the shared architecture between PolD DP1 and Homo sapiens Polδ B-subunit (PDBid: 3EOJ (ref. 26 )). Top panels show the electrostatic potentials of DP1 and Polδ OB domains mapped on their solvent-accessible surface at contouring ±5 kT e −1 . The potential was calculated with APBS [64] . Full size image Alteration of the canonical oligonucleotide-binding surface of their OB domain and inactivation of catalytic nuclease motifs of their PDE domain suggest that eukaryotic DNAP B-subunits have been evolutionary converted to a scaffold mainly responsible for their multi-subunit assembly and perhaps allosteric regulation. Taking into account that B-subunits are indispensable components of all replicative B-family DNAPs and that there is a significant sequence similarity between the C-terminal Zn finger of Polɛ and of PolD DP2, it has been suggested that DP2 is a highly divergent homologue of B-family DNAPs [31] . However, the DP2 structure shares no similarity with known structure of DNAPs, including family-B DNAPs, thereby formally invalidating this hypothesis, as shown below. Structure of DP2 DNAP catalytic subunit The DP2 structure reveals an extended molecule with overall dimensions of 55 × 60 × 110 Å 3 and four domains: the N-terminal domain (NTD; residues 1–285), the central domain (residues 308–667), the catalytic domain (residues 668–996) and a fragment of the CTD (residues 997–1,039) ( Fig. 1b ). The most prominent feature of the DP2 architecture is the extensive interaction between the NTD and catalytic domain, which results in a wide interfacial crevice that hosts the DNAP active site, formed by two double-psi β-barrels (DPBBs). Unexpectedly, PolD DP2 and ‘two-barrel’ RNA polymerases (RNAPs) share a conserved architecture in their active sites. The NTD structure shows a 45-residue long N-terminal extension dedicated to interaction with the catalytic domain ( Fig. 1b ). This N-terminal extension, named here ‘N-terminal self-assembly region’, consists of a long α-helix (α 1 ) and a short β-strand (β 1 ) that brings together the NTD and catalytic domains through a large interface of 1,700 Å 2 buried surface area. The majority of the interactions with the catalytic domain are mediated by helix α 1 and the α 1 –β 1 connecting loop, which fit within a long and shallow groove formed at the surface of the catalytic domain ( Fig. 4a ). The chemical nature of this interaction is diverse ( Fig. 4b,c ) and includes polar contacts, extensive van der Waals contacts between hydrophobic residues, as well as secondary structure interactions between two β-strands, β 1 (NTD) and β 33 (catalytic domain). DP2 structure allows a rationalization of previous biochemical studies indicating an intrasubunit interaction between the N terminus and C terminus of the P. horikoshii DP2 subunit [10] , [14] . The rest of the NTD structure shows a compact α/β structure that consists of a twisted β-sheet (β 2 –β 4 ) and 10 α-helices (α 2 –α 11 ). The P. abyssi NTD shares a strong similarity with the P. horikoshii DP2 (50–290) structure (r.m.s.d. 0.463 Å calculated over 241 Cα) that was exploited at the initial phase of model building (see Methods). Interestingly, the N-terminal self-assembly region was not ordered in the P. horikoshii isolated PolD NTD structure, consistent with its dedication to interaction with the catalytic domain. 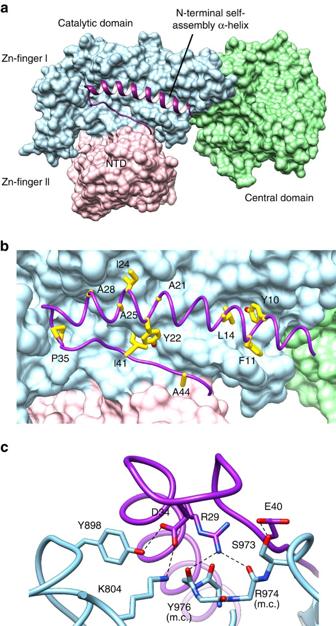Figure 4: Interactions within the DP2 N-terminal self-assembly region and the catalytic domain. (a) Overall view highlighting the involvement of the N-terminal self-assembly α-helix with the catalytic domain. The N-terminal self-assembly α-helix is depicted as purple ribbon, the NTD and catalytic domains as a molecular surface in pink and blue, respectively. (b) Hydrophobic interactions at the N-terminal α-helix/catalytic domain interface. Important hydrophobic side chains are shown as yellow sticks. (c) Close-up view of the hydrophilic interactions within the N-terminal self-assembly α-helix and the catalytic domain. Side chains are drawn as sticks and hydrogen bonds as dashed lines. Figure 4: Interactions within the DP2 N-terminal self-assembly region and the catalytic domain. ( a ) Overall view highlighting the involvement of the N-terminal self-assembly α-helix with the catalytic domain. The N-terminal self-assembly α-helix is depicted as purple ribbon, the NTD and catalytic domains as a molecular surface in pink and blue, respectively. ( b ) Hydrophobic interactions at the N-terminal α-helix/catalytic domain interface. Important hydrophobic side chains are shown as yellow sticks. ( c ) Close-up view of the hydrophilic interactions within the N-terminal self-assembly α-helix and the catalytic domain. Side chains are drawn as sticks and hydrogen bonds as dashed lines. Full size image The catalytic domain is composed of a central six-stranded DPBB (β 25 and β 28–32 ) ( Fig. 1b ). The first (β 25 ) and second (β 28 ) β-strands of the DPBB are connected by a 40-residue-long insertion, which forms a compact structure composed of two short β-strands (β 26–27 ) and two short α-helices (α 28–29 ) that interact with the central domain. The peptide chain connecting the fifth (β 31 ) and the sixth (β 32 ) β-strands of the barrel forms a right-handed α-helix followed by a 10-residue-long loop, which constitutes the most conserved sequence motif of DP2 ( Supplementary Fig. 7 ). This motif comprises two invariant aspartic residues (D961 and D963), which were previously shown to be catalytically critical for PolD DNAP activity [32] . The DPBB is preceded by a helical region composed of three α-helices (α 24 , α 26–27 ) and a tandem repeat of two zinc modules, named Zn-I and Zn-II. The coordinating metals were confidently assigned to zinc by observing strong peaks in the anomalous maps using diffraction data collected at the Zn K-edge, that disappear below this edge ( Supplementary Fig. 8 ). In both cases, Zn 2+ are tetrahedrally coordinated by two pairs of cysteines located in turns, but apart from that the two zinc-binding modules bear no structural relationship to each other. In particular, zinc module Zn-II has a short helix insertion, an uncommon structural feature shared only with the zinc-binding module of the large subunit of the human transcription factor II-E [33] . While the N-terminal and catalytic domains interact extensively, the rest of the DP2 structure folds into a central domain that shares a relatively modest 460 Å 2 interaction surface region with the other domains ( Fig. 1b ). This results in an increased flexibility of the interfacial region between the central domain and the rest of the protein. As a consequence of this flexibility, several fragments of the peptide chains, all located within this interfacial region, were not modelled due to a lack of interpretable electron density. In particular, the peptide chains connecting the NTD to the central domain (residues 286–307), strands β 7 to β 8 (residues 358–364), strands β 8 to β 9 (residues 376–392) and strand β 18 to the catalytic domain (residues 654–668) were not visible in the electron density. This complicated the assignment of a second DPBB subdomain, which faces the first one located in the catalytic domain. Indeed, only five out of six strands (β 7–9 , β 13 and β 18 ) composing this second DPBB have been modelled. To conform to the canonical topology of DPBB, the missing strand should be located in a stretch of 17 missing residues (376–392), which connect the β 8 and β 9 strands of the DPBB. Consistently, secondary structure predictions [34] suggest that this peptide indeed contains a β-strand ( Supplementary Fig. 7 ). The two DPPB subdomains located in the central domain, and the catalytic domain of the DP2 structure are, respectively, named DPBB-1 and DPBB-2, according to their order of occurrence in the primary structure. The location of the two DPBB, with respect to each other, is very similar to that observed in ‘two-barrel’ RNAPs (see below). Owing to the presence of several insertions DPBB-1 is spread throughout the central domain that also contains a seven-stranded antiparallel β-sheet (β 10–12 and β 14–17 ) wrapped around by two helices (α 13–14 ) from one side and by four helices (α 19–22 ) from the other side. This β-sheet is itself interrupted by a small α-helical region formed by four helices (α 15–18 ). The CTD of DP2 (1,000–1,270) is known to be dedicated to an interaction with the DP1 subunit [13] , [14] . For solubility and crystallization purposes, the CTD was truncated by 220 residues (1,051–1,270). The 50 residues of the CTD present in our construct (1,000–1,050) are partly disordered, except for two helices α 32 and α 33 (residues 1,011–1,039), which bind next to the interface between the central and catalytic domains through interactions with the DPPB-1 and helix α 32 . This partial structure of the CTD suggests however that the 3′–5′ proofreading DP1 subunit might be localized next to the polymerase active site. Evolutionary relationship between PolD and two-barrel RNAPs When DP2 structure was compared with structures in Protein Data Bank, no significant structural similarity with known DNAP was detected. Instead, PolD shares an unexpected structural homology with the ‘two-barrel’ family of RNAP [35] ( Supplementary Fig. 9 ), which includes multi-subunit transcriptases from all domains of life, homodimeric RNA-silencing pathway RNAPs and atypical RNAPs encoded by some viruses, including some bacteriophages [36] . However, only the DPBB-2 domain was detected by Dali [25] and the other one, DPBB-1, could only be detected manually. Two-barrel RNAPs share a common catalytic centre that is formed between two DPBBs (here after called DPBB-A and DPBB-B), which contribute distinct amino-acid residues to the active site in an asymmetrical fashion [35] , [37] , [38] . DPBB-A contains a DFDGDE signature [37] , whose aspartate carboxylate residues chelate catalytic Mg 2+ ions, and DPBB-B contributes two lysine residues that are involved in DNA binding. Both DPBB subdomains of ‘two-barrel’ RNAPs show a remarkable degree of three-dimensional similarity to those of PolD DP2 ( Fig. 5a,b ). Even in the absence of substrate and Mg 2+ ions, the catalytic loop in the DPBB-2 of PolD structure can be superposed with the DPBB-A RNAP minimal core structures with a significant overlap ( Fig. 3b ). In particular, the two mandatory aspartic residues of PolD are conserved and aligned with two out of three canonical catalytic aspartic residues in multi-subunit RNAP ( Fig. 5c ). Although lacking one β-strand located within a fragment of 17 missing residues, the DPBB-1 domain of PolD structure can also be superposed with the DPBB-B of RNAP. In Saccharomyces cerevisiae RNAP-II structure [39] , the corresponding region contains two conserved lysine residues (K979 and K987 in RPB1 subunit), whose side chains point towards the active site and are involved in DNA binding. A multiple-sequence alignment of the corresponding 17 missing residues in PolD structure shows the presence of three basic residues, two lysines (K386 and K392) and one arginine (R389), all located within a highly conserved sequence motif ( Supplementary Fig. 7 ). These conserved positively charged residues might occupy a location similar in PolD to that observed in their RNAP counterparts and therefore contribute to DNA binding. 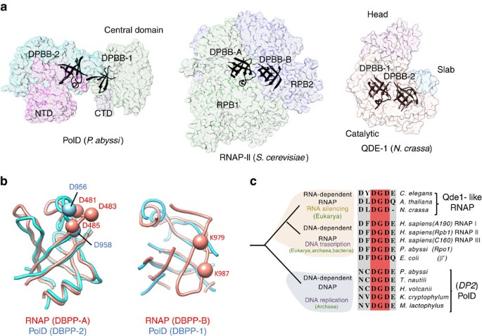Figure 5: Shared active site architecture between PolD DP2 and ‘two-barrel’ RNAPs. (a) Overview of the conserved ‘two-barrel’ catalytic core in PolD DP2,S. cerevisiaeRNAP-II (PDBid: 4BBS (ref.39)) andNeurospora crassaQDE-1 (PDBid: 2J7O (ref.41)). (b) Superposition of the DPBB subdomains of PolD (blue) andS. cerevisiaeRNAP-II (pink). Left: the PolD DPBB-II subdomain is superimposed on the RNAP-II DPBB-A subdomain (Cα r.m.s.d. of 1.72 Å calculated over 73 residues). Cα of the catalytic aspartate residues are shown as spheres. Right: the PolD DPBB-I subdomain is superimposed on the RNAP-II DPBB-B subdomain (Cα r.m.s.d. of 2.21 Å calculated over 42 residues). (c) Possible evolutionary relationship between the DNA-dependent DNAP PolD, DNA-dependent RNAPs and RNA-dependent RNAPs. Conserved catalytic motifs are highlighted in a multi-sequence alignment. The alignment was generated using representative protein with a large sequence diversity to illustrate sequence variability (GI accession number): (i) for RNA-dependent RNAPsCaenorhabditis elegans(392,886,219),Arabidopsis thaliana(42,569,168) andN. crassa(85,091,735); (ii) for DNA-dependent RNAPsHomo sapiens(4,096,591; 119,610,588; 20,159,751),Pyrococcus abyssi(499,169,463) andEscherichia coli(983,454,941); and (iii) for D-family DNAPsP. abyssi(504,648,395),Thermococcus nautili(757,137,858),Haloferax volcanii(490,144,762),Korarchaeum cryptofilum(501,267,152) andMethanosarcina mazei(814,797,709). Figure 5: Shared active site architecture between PolD DP2 and ‘two-barrel’ RNAPs. ( a ) Overview of the conserved ‘two-barrel’ catalytic core in PolD DP2, S. cerevisiae RNAP-II (PDBid: 4BBS (ref. 39 )) and Neurospora crassa QDE-1 (PDBid: 2J7O (ref. 41 )). ( b ) Superposition of the DPBB subdomains of PolD (blue) and S. cerevisiae RNAP-II (pink). Left: the PolD DPBB-II subdomain is superimposed on the RNAP-II DPBB-A subdomain (Cα r.m.s.d. of 1.72 Å calculated over 73 residues). Cα of the catalytic aspartate residues are shown as spheres. Right: the PolD DPBB-I subdomain is superimposed on the RNAP-II DPBB-B subdomain (Cα r.m.s.d. of 2.21 Å calculated over 42 residues). ( c ) Possible evolutionary relationship between the DNA-dependent DNAP PolD, DNA-dependent RNAPs and RNA-dependent RNAPs. Conserved catalytic motifs are highlighted in a multi-sequence alignment. The alignment was generated using representative protein with a large sequence diversity to illustrate sequence variability (GI accession number): (i) for RNA-dependent RNAPs Caenorhabditis elegans (392,886,219), Arabidopsis thaliana (42,569,168) and N. crassa (85,091,735); (ii) for DNA-dependent RNAPs Homo sapiens (4,096,591; 119,610,588; 20,159,751), Pyrococcus abyssi (499,169,463) and Escherichia coli (983,454,941); and (iii) for D-family DNAPs P. abyssi (504,648,395), Thermococcus nautili (757,137,858), Haloferax volcanii (490,144,762), Korarchaeum cryptofilum (501,267,152) and Methanosarcina mazei (814,797,709). Full size image The finding that PolD and ‘two-barrel’ RNAPs share a common catalytic core with similar sequence motifs considerably extends the ‘two-barrel’ RNAPs protein family and links it, for the first time, with the DNAPs. Our study also shows that the -DFDGDE- motif is not as strict as previously thought ( Fig. 5c ) and show that PolD constitute another example of a ‘two-barrel’ polymerase that carries the two DPBB domains on the same polypeptide chain, as previously observed on QDE-1, an RNAP that synthesizes siRNA in plants [40] , [41] ( Fig. 5a ). The ‘two-barrel’ architecture defines the DP2 catalytic site In addition to their structural similarity with the catalytic core of two-barrel RNAPs, converging observations suggest that the DPBB subdomains of PolD host the DNAP active site. Indeed, the peptide chain connecting the fifth (β 31 ) and the sixth (β 32 ) β-strands of the DPBB-2 comprises two invariant aspartic residues (D956 and D958), which were previously shown to be critical for DNAP catalytical activity, following an extensive alanine-scan site-directed mutagenesis study of all aspartate residues of DP2 (ref. 32 ). In addition, alteration of the α-helix that precedes these catalytic residues markedly reduced DNA-binding ability and protein stability [42] . Interestingly, in several species including P. abyssi , the catalytic loop contains an intein insertion site, which is known to be often located in motifs important for enzymatic activities, especially in archaeal DNA replication proteins [43] . The catalytic loop is solvent-exposed and located within a 55-Å long and 25-Å wide crevice, whose dimensions are ideally suited to orient a 1.5 helical turn long (about 15 bp) duplex B-DNA within the active site. The crevice exposes residues that display a high degree of conservation relative to the rest of the solvent-exposed regions ( Fig. 6a ). In addition, the electrostatic potential surface of the PolD DP2 subunit presents a highly biased distribution of positively charged residues, located along an arch running from the catalytic loop to the two zinc-binding modules, which could interact with the phosphate backbone of template DNA ( Fig. 6b ). The crevice is located at the interface between the NTD and catalytic domains, thereby highlighting the functional implications of this inter-domain interaction for DNAP function. Consistently, former biochemical assays revealed that disrupting the N-terminal self-assembly α-helix of P. abyssi PolD reduces DNAP processivity [44] . 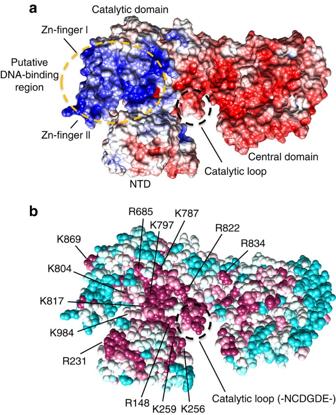Figure 6: Structural features of PolD DP2 active site. (a) Electrostatic potential of DP2, mapped on its solvent-accessible surface at contouring of ±5 kT e−1. Positive potential is in blue, negative charge in red. The potential was calculated with APBS64. (b) Amino-acid conservation mapped on the crystal structure of DP2. The evolutionary conservation analysis of surface residues was performed with the ConSurf66server, based on 12 evolutionary-distant sequences of DP2. Degree of conservation is shown by colour range, from magenta (highest conservation) to cyan (lowest). The structure is shown in space fill representation. Highly conserved residues that might be important for the functional role of DP2 are numbered. Figure 6: Structural features of PolD DP2 active site. ( a ) Electrostatic potential of DP2, mapped on its solvent-accessible surface at contouring of ±5 kT e −1 . Positive potential is in blue, negative charge in red. The potential was calculated with APBS [64] . ( b ) Amino-acid conservation mapped on the crystal structure of DP2. The evolutionary conservation analysis of surface residues was performed with the ConSurf [66] server, based on 12 evolutionary-distant sequences of DP2. Degree of conservation is shown by colour range, from magenta (highest conservation) to cyan (lowest). The structure is shown in space fill representation. Highly conserved residues that might be important for the functional role of DP2 are numbered. Full size image The DNAP active site shows an increased flexibility compared with the rest of the protein. Some of the conserved motifs in the DPBB-1 subdomain are not seen in the electron density map of the DP2 structure. Comparison with ‘two-barrel’ RNAPs suggests that these disordered conserved motifs in DP2 structure also contain important catalytic residues, including basic residues that may be involved in DNA binding (see above). The increased flexibility of catalytic residues might be reflected by the fact that the DP2 structure shows no Mg 2+ bound in the active site, while structures of ‘two-barrel’ RNAPs usually do. The flexibility observed in the active site of DP2 structure might be due to the absence of the DNA substrate, or to the CTD truncation of the DP2 (1–1,050) construct used in this study. Alternatively, the region of the active site might be stabilized on interaction with the DP1 subunit, as suggested by biochemical assays showing that DNAP activity is stimulated on association of the two PolD subunits [7] , [13] , [14] . Additional studies, including solving a substrate-bound structure of PolD, are required to establish the molecular details of DNA binding, nucleotide selectivity, polymerization and decipher the specificities of D-family DNAPs compared with other DNAP families. DNAPs have been the subject of extensive structural biology research for decades, which resulted in high-resolution structures of representative DNAPs belonging to different families, following the pioneer work on Klenow fragment of Escherichia coli DNA PolI (ref. 45 ). Up to now, DNAPs of known structures could be divided into two groups based on the structural fold of their catalytic sites [24] . The first group assembles DNAPs that structurally resemble the E. coli PolI Klenow-fold [46] , often referred as right-handed polymerases [2] . Their overall fold is characterized by thumb, fingers and palm subdomain, and is shared by A-/B-/Y-family DNAPs, reverse transcriptases and telomerases [47] . The second group, often referred to as Polβ-like polymerases, includes X- and C-families DNAPs, and shares a similar three-dimensional arrangement of catalytic aspartates in the active site [48] , [49] and a two-metal-ion mechanism [50] with the first group but has a completely different topology in the palm subdomain ( Fig. 7 ). In many aspects, crystal structures of both DP1 and DP2 subunits revealing that PolD is an atypical DNAP, change this view by linking together DNAP and RNAP. A third group of nucleotide polymerases is created, whose members can perform DNA-dependent RNA or DNA synthesis, and RNA-dependent RNA synthesis. 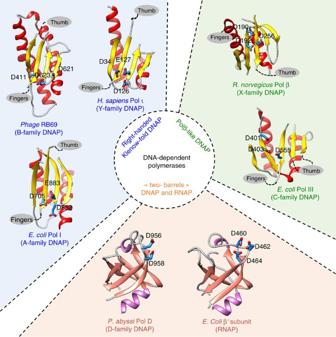Figure 7: An updated structural classification of all DNA-dependent polymerases. The following crystal structures were used: Polβ fromRattus norvegicus(PDBid: 1BPB), Pol III fromEscherichia coli(PDBid: 2HNH), Polι fromHomo sapiens(PDBid: 1T3N), PolB fromEnterobacteria phage RB69(PDBid: 1IH7), Pol I fromE. coli(PDBid: 1KLN), RNAP β′ subunit fromE. coli(PDBid: 4MEX) and PolD fromP. abyssi(this study). Figure 7: An updated structural classification of all DNA-dependent polymerases. The following crystal structures were used: Polβ from Rattus norvegicus (PDBid: 1BPB), Pol III from Escherichia coli (PDBid: 2HNH), Polι from Homo sapiens (PDBid: 1T3N), PolB from Enterobacteria phage RB69 (PDBid: 1IH7), Pol I from E. coli (PDBid: 1KLN), RNAP β′ subunit from E. coli (PDBid: 4MEX) and PolD from P. abyssi (this study). Full size image First, DP1 subunit contains a calcineurin-like phosphodiesterase fold that is responsible for the 3′–5′ proofreading exonuclease activity. In one way, this clearly links PolD to the DNAP world because this fold is present—but catalytically inactive—in the regulatory B-subunit of eukaryotic DNAP. However, in most other structurally characterized DNAPs the catalytically active proofreading domains fold into an α/β structure with a twisted five-stranded mixed β-sheet [51] , [52] , [53] , which shares no structural homology with DP1. While calcineurin-like phosphoesterases includes a diverse range of phosphoesterases [54] , including protein phosphoserine phosphatases, nucleases, nucleotidases, sphingomyelin phosphodiesterases and 2′–3′ cAMP phosphodiesterases, their dedication to DNA proofreading is unique to PolD. Among the calcineurin-like superfamily of proteins, DP1 shows the highest structural similarity with the DNA repair exo-/endonuclease Mre11. Catalytic motifs are remarkably conserved among both enzymes suggesting that they share a common hydrolase catalytic mechanism. However, comparison of DP1 and P. furiosus Mre11 dAMP-bound structure [19] revealed substantial differences in the way the adenine base fits into the active site that may reflect the differences in specificity between both nucleases. In particular, the DP1 active site seems shaped to favour binding of mispaired 3′-terminal nucleotide over paired 3′-terminal nucleotide, a property that is expected for a DNAP-associated proofreading exonuclease. In addition, the dinuclear Fe 3+ /Zn 2+ metal centre observed in DP1 is another specificity of the PolD structure. Indeed, while asymmetric dinuclear Fe 3+ /Zn 2+ catalytic centres are common among calcineurin-like phosphoesterases, they are uncommon among nucleases, which prefer symmetrical dinuclear metal centres (Mg 2+ , Mn 2+ and Zn 2+ ) [55] . Second, the structure of DP2 catalytic subunit shows that it shares no significant structural similarity with known DNAP. Instead, PolD DP2 shares an unexpected structural homology with the ‘two-barrel’ family of RNAP [35] , which includes multi-subunit transcriptases from all domains of life, homodimeric RNA-silencing pathway RNAPs and atypical RNAPs encoded by some viruses and phages [36] . The finding that PolD and ‘two-barrel’ RNAPs share a common catalytic core with similar sequence motifs considerably extends the ‘two-barrel’ RNAPs protein family and links it with the DNAPs ( Fig. 7 ). Also, it shows that the two DPBB subdomains can be part of the same polypeptide chain, contrary to most RNAPs (with the exception of siRNA synthesizing QDE-1 RNAP). This defines a novel paradigm for the classification and possible evolutionary relationships between different types of both RNA and DNAPs. It bridges together, for the first time in the non-viral world, DNA transcription and DNA replication within the same protein superfamily, suggesting that these distantly related polymerases share a common ancestor, which might have been selected for nucleotide polymerization in early forms of life. The capacity of PolD to use RNA-primed DNA might be a property inherited from its common ancestor to RNAP [7] . However, the exact evolutionary history of ‘two-barrel’ polymerases remains at this stage speculative, especially as other ‘two-barrel’ RNAPs that are found in some large DNA viruses (baculoviruses and nucleocytoplasmic large DNA viruses, including mimiviruses [35] ), are very different from their cellular homologues. Finally, PolDs encoded from Thermococcales possess high processivity, specificity and thermostability properties that confer them a biotechnological potential [56] , which has remained unexploited up to now due to the lack of detailed structural information. The new structures described here pave the way to the complete description of the molecular mechanisms of DNA binding, nucleotide selection and proofreading of this new family of DNAPs that might lead to variants of PolD with better PCR or sequencing properties. Cloning and protein purification Residues 144–622 of P. abyssi DP1 and residues 1–1,051 of P. abyssi DP2 were cloned into an RSF1-Duet expression vector (Novagen) fused to an N-terminal 14-histidine tag. The protein was expressed by 1 mM isopropyl- D -thiogalactoside induction in E. coli strain BL21(DE3) Rosetta2 grown overnight in LB (Lysogeny Broth) at 20 °C and purified by Ni-NTA and heparin chromatography (GE Healthcare), followed by TEV cleavage of the tag and size-exclusion chromatography. The purified DP1 protein was concentrated to 3 mg ml −1 in 20 mM Tris HCl pH 8, 200 mM NaCl, 5% glycerol. The purified DP2 protein was concentrated to 10 mg ml −1 in 20 mM Tris HCl (pH 7.5) and 50 mM NaCl. Both purified proteins were flash frozen in liquid nitrogen and stored at −80 °C. Biochemical 3′–5′ exonuclease and primer-elongation assays Oligonucleotides Nucleotide sequences of the DNA substrates were inspired by Jokela et al . [24] . A 27mer DNA primer with three non-complementary bases at its 3′-end was used in the exonuclease assays (5′-ACGCCAGGCTTCGCCAGTCACGAT ACT -3′). A 24mer DNA primer was used in the DNAP primer-extension assays (5′-ACGCCAGGCTTCGCCAGTCACGAC-3′). The same 60mer DNA template was used in both reactions (5′-GCGGACTGCGATCGTACCTACGGACCTGCAGCTGACGTCGTGACTGGCGAAGCCTGGCGT-3′). 32 P-labelling DNA primers were 5′-labelled with 32 P using T4 polynucleotide kinase (PNK). A unit of 20 μM DNA was incubated for 1 h at 37 °C with 10 U PNK (Thermo scientific) and 100 μCi γ- 32 P-labelled ATP. The labelling reaction was stopped by heating the sample at 70 °C for 10 min. DNA duplex annealing A unit of 40 μM template was mixed with 40 μM labelled primer, annealing buffer (20 mM Tris-HCl (pH 8), 10 mM MgCl 2 and 1 mM EDTA) and incubated for 5 min at 95 °C. Activity tests DP1: 10 μM DP1(144–622), 50 nM DNA duplex, 25 mM Tris-HCl pH7.6, 25 mM NaCl and 2 mM MgCl 2 were incubated at 55 °C for 10, 45, 90 and 150 s. DP2: 50 nM DNA duplex was incubated at 55 °C with 25, 35 or 50 μM DP2(1–1,061) for 1, 5 or 10 min, in presence of 200 nM dNTPs and NEB 2.1 reaction buffer (New England Biolabs). All reactions were stopped by adding formamide. Samples were run through a 15% acrylamide–8 M urea sequencing gel and revealed using a PhosphorImager Storm 860 (Fujifilm). Crystallization DP1 was crystallized by hanging-drop vapour diffusion at 4 °C, mixing 1 μl of protein (3 mg ml −1 ) with 1 μl of crystallization buffer containing 100 mM sodium cacodylate, pH 6.7, 200 mM calcium acetate and 2–6% PEG 8000. Crystals of DP1 bound to dAMP were obtained by co-crystallization in presence of 5 mM dAMP. DP2 was crystallized by sitting-drop vapour diffusion at 18 °C, mixing 1 μl of protein (10 mg ml −1 ) with 1 μl of crystallization buffer containing 60 mM MES, pH 5.6, 300 mM sodium chloride and 6% PEG 6000. Both DP1 and DP2 crystals were optimized using micro-seeding from a solution of crushed crystals. DP1 and DP2 crystals were cryo-cooled with 35% and 27.5% ethylene glycol, respectively. For the purpose of phasing (see below), DP1 and DP2 crystals were soaked overnight in a solution containing 5 mM K 2 Pt(NO 2 ) 4 (Jena Bioscience). Phasing and structure determination DP1 . Platinum-derived crystals diffracted up to 2.8 Å on Proxima 2 (SOLEIL, Gif-sur-Yvette, France). The dAMP-bound DP1 crystals diffracted up to 2.5 Å on ID23-1 (ESRF, Grenoble, France). The crystal structure was determined with phase information using PHENIX [57] derived from anomalous scattering data collected at the Pt L-III edge (eight sites, figure-of-merit 0.45). The crystals belonged to the P2 1 2 1 2 1 space group with two copies of the protein in the asymmetric unit. An initial model was obtained using PHENIX [57] , completed manually in Coot [58] and refined in Buster [59] . For details, see Table 1 . DP2: platinum-derived crystals diffracted up to 3.1 Å on Proxima 1 (SOLEIL, Gif-sur-Yvette, France). Native DP2 crystals diffracted up to 2.2 Å on ID23-1 (ESRF, Grenoble, France). Initial phases were derived using PHENIX [57] from anomalous scattering data collected at the Pt L-III edge (nine sites, figure-of-merit 0.40). The crystal structure of the NTD (48–291) of P. horikoshii DP2 subunit (PDBid: 3,059 (ref. 10 )) was fitted in the electron density on superposition to the initial model generated by AutoBuild [57] . Subsequent rounds of phase combination and automatic model building were notably improved. The crystals belong to the P2 1 2 1 2 1 space group with one copy of the protein in the asymmetric unit. The model was then built manually in Coot [58] . For details, see Table 1 . Table 1 Data collection and refinement statistics. Full size table Model building and data refinement DP1 . The final model was refined in Buster to R / R free values of 19.7/22.5 at 2.5 Å resolution. Non-crystallographic symmetry restraints were used throughout refinement, with one TLS parameter per molecule. Residues 144–151, 164–173, 213–224 and 514–517 (only in chain B), which were not visible in the electron density, were not included in the final model. One dAMP molecule and 66 water molecules were added per monomer. In the final electron density, remaining peaks that could not be attributed to water were modelled with acetate, ethylene glycol and three calcium ions, which were present in the crystallization solution (see above). The active site includes two tightly bound metal ions, zinc and iron, whose presence was confirmed by collecting anomalous data at the zinc and iron K-edges (see below and Supplementary Fig. 2 ). Of all residues, 96.2% were in the favoured regions of the Ramachandran plot with three outliers. Two out of these three outliers correspond to His residues that participate to metal ion coordination and are located in the active site in a region where the electron density is clearly defined. Metal ion coordination causes a subtle distortion of the backbone resulting with these residues being Ramachandran outliers. The Molprobity [60] score for the refined model is 1.60, in the 99th percentile of structures refined at comparable resolution. DP2: the final model was refined in Buster to R / R free values of 19.9/23.5 at 2.2 Å resolution, with five TLS parameters (defined using the TLSMD [61] web server) for the protein chain. Residues 1–3, 286–307, 325–338, 358–363, 376–392, 654–667, 1,000–1,010 and 1,041–1,061, which were not visible in the electron density were not included in the final model. Those residues are concentrated in a region that connects the NTD to the central domain. These residues are highly divergent between PolDs from different species. To gain confidence in the assignment of the sequence of the protein within regions where the chain is not continuous, we collected an additional anomalous data set at the sulphur edge (1.8 Å). Taking advantage of the 10 cysteines and 14 methionines of the protein, we confirmed the correctness of sequence assignment. In all, 242 water molecules and 2 zinc ions (see below and Supplementary Fig. 7 ) were added to the model. Of all residues, 97.4% were in the favoured regions of the Ramachandran plot with no outliers. The Molprobity [60] score for the refined model is 1.43, in the 99th percentile of structures refined at comparable resolution. The quality of the electron density is illustrated in Supplementary Fig. 10 . Assigning transition metal ions identities DP1 . The active site of DP1 contains His, Asp and Asn residues, which are conserved within the phosphodiesterase protein superfamily and coordinate tightly two catalytic metal ions. The Fourier Fo–Fc difference electron density map shows two strong peaks at 12 σ in the active site of DP1, consistent with the presence of two metal ions. An X-ray fluorescence scan on DP1 crystals detected the presence of three transition metal ions: zinc, iron and calcium. While calcium is present in the crystallization solution (see above), neither iron nor zinc ions were introduced in purification or crystallization buffers. To assign the identity of the two metal ions in the active site of DP1 (arbitrarily named sites A and B), we collected four anomalous data sets: the first one at the iron K-edge (1.7394 Å), the second one right below the iron K-edge (1.7557 Å), the third one at the zinc K-edge (1.2815 Å) and the fourth one right below the zinc K-edge (1.2881 Å) ( Supplementary Fig. 2 ). All data sets were collected on different regions of the same crystal. The anomalous map calculated from the data set collected at the iron K-edge shows two peaks: a stronger peak at site A (10.5 σ ), a weaker peak at site B (7.6 σ ). The peak at site A is lost in the anomalous map calculated from the data set collected below the iron K-edge, thereby showing that iron ions specifically binds at site A. The anomalous map calculated from the dataset collected at the zinc K-edge shows two closely equivalent peaks at site A (10.2 σ ) and at site B (8.9 σ ). Both peaks are substantially lower in the anomalous map calculated from the data set collected below the zinc K-edge (5.1 σ ), suggesting that zinc ions bind to both sites. Overall, this set of experiments shows that iron ion binds mainly to site A, zinc ions to both A and B sites. In the final model, site A and B were modelled with iron and zinc ions, respectively, in line with other calcineurin-like phosphodiesterases, which show dual binding of zinc and iron ions within their active site: for example, mammalian calcineurin [15] (PDBid 1TCO) and the red kidney bean purple acid phosphatase [16] (PDBid 1KBP). DP2: the final model includes two metal-binding motifs, each coordinated by four cysteine ligands. To confirm the presence of zinc within these motifs, we collected two anomalous data sets: the first one at the zinc K-edge (1.2820 Å), the second one right below the zinc K-edge (1.2882 Å). While the anomalous map calculated from the data set collected at the zinc K-edge shows two strong peaks (17 σ for zinc I, 9 σ for zinc II), the anomalous map calculated from the data set collected below the zinc K-edge shows no such peaks, thereby confirming the presence of zinc in both sites ( Supplementary Fig. 8 ). Structure analysis Dali [25] was used to compare the DP1 and DP2 structures with those of the Protein Data Bank. The programme Superpose implemented in CCP4 (ref. 62 ) was used for structural alignments and Areaimol [63] for accessible surface area measurements (CCP4). Electrostatic surface potentials were calculated using APBS [64] in Chimera [65] . The evolutionary conservation analysis of surface residues was performed with the Consurf [66] server. Figures were prepared with Chimera [65] and PyMOL (The PyMOL Molecular Graphics System, Version 1.8 Schrödinger, LLC.). Data availability Coordinates and structure factors for DP1 and DP2 crystal structures were deposited in the Protein Data Bank under the accession codes 5IHE and 5IJL , respectively. All other data are available in the manuscript and associated materials, or from the authors on reasonable request. How to cite this article: Sauguet, L. et al . Shared active site architecture between archaeal PolD and multi-subunit RNA polymerases revealed by X-ray crystallography. Nat. Commun. 7:12227 doi: 10.1038/ncomms12227 (2016).